Reconstructing propagation networks with natural diversity and identifying hidden sources Our ability to uncover complex network structure and dynamics from data is fundamental to understanding and controlling collective dynamics in complex systems. Despite recent progress in this area, reconstructing networks with stochastic dynamical processes from limited time series remains to be an outstanding problem. Here we develop a framework based on compressed sensing to reconstruct complex networks on which stochastic spreading dynamics take place. We apply the methodology to a large number of model and real networks, finding that a full reconstruction of inhomogeneous interactions can be achieved from small amounts of polarized (binary) data, a virtue of compressed sensing. Further, we demonstrate that a hidden source that triggers the spreading process but is externally inaccessible can be ascertained and located with high confidence in the absence of direct routes of propagation from it. Our approach thus establishes a paradigm for tracing and controlling epidemic invasion and information diffusion in complex networked systems. One of the outstanding problems in interdisciplinary science is nonlinear and complex systems identification, prediction and control. Given a complex dynamical system, the various types of dynamical processes are of great interest. The ultimate goal in the study of complex systems is to devise practically implementable strategies to control the collective dynamics. A great challenge is that the network structure and the nodal dynamics are often unknown but only limited measured time series are available. To control the system dynamics, it is imperative to be able to map out the system details from data. Reconstructing complex network structure and dynamics from data, the inverse problem, has thus become a central issue in contemporary network science and engineering [1] , [2] , [3] , [4] , [5] , [6] , [7] , [8] . There are broad applications of the solutions of the network reconstruction problem, due to the ubiquity of complex interacting patterns arising from many systems in a variety of disciplines [9] , [10] , [11] , [12] . An important class of collective dynamics is epidemic spreading and information diffusion in the human society or on computer networks [13] , [14] , [15] , [16] , [17] , [18] , [19] , [20] . The past decades have witnessed severe epidemic outbreaks at the global scale due to the mutation of virus, including SARS [21] , [22] , H5N1 (refs 23 , 24 ), H1N1 (refs 25 , 26 ) and the recent invasion of H7N9 in eastern China [27] , [28] . Our goal is to reconstruct the networks hosting the spreading process and identify the source of spreading using limited measurements. This is especially challenging due to (1) difficulty in predicting and monitoring mutations of deadly virus and (2) absence of epidemic threshold in heterogeneous networks [29] , [30] , [31] , [32] . Another example is rumour propagation in the online virtual communities, which can cause financial loss or even social instabilities, such as the 2011 irrational and panicked acquisition of salt in southeast Asian countries caused by the nuclear leak in Japan. In this regard, identifying the propagation network for controlling the dynamics is of great interest. Another significant challenge in reconstructing a spreading network lies in the nature of the available time series: they are polarized, despite stochastic spreading among nodes. Indeed, the link pattern and the probability of infection are encrypted in the binary status of individuals, infected or not, analogous to the collapse of wave function to one associated with some discrete quantum state induced by observation in quantum mechanics. There have been recent efforts in addressing the inverse problem of some special types of complex propagation networks [33] , [34] . In particular, for diffusion process originated from a single source, the routes of diffusion from the source constitute a tree-like structure. If information about the early stage of the spreading dynamics is available, it would be feasible to decode all branches that reveal the connections from the source to its neighbours, and then to their neighbours and so on. Taking into account the time delays in the diffusion process enables a straightforward inference of the source in a complex network through enumerating all possible hierarchical trees [33] , [34] . However, if no immediate information about the diffusion is available, the tree-structure-based inference method is inapplicable, and the problem of network reconstruction and locating the source becomes extremely challenging, hindering control of diffusion and delivery of immunization. The loss of knowledge about the source is common in real situations. For example, passengers on an international flight can carry a highly contagious disease, making certain airports the immediate neighbours of the hidden source, which would be difficult to trace. In another example, the source could be migratory birds coming from other countries or continents. A general data-driven approach, applicable in such scenarios, is still lacking. In this paper, we develop a general theoretical framework to reconstruct complex propagation networks from time series based on the compressed sensing theory (CST) [35] , [36] , [37] , [38] , [39] , [40] , a novel optimization paradigm for sparse-signal reconstruction with broad applications in signal and image processing. Owing to the striking characteristics of CST such as the extremely low data requirement and rigorous guarantee of convergence to optimal solutions, our framework is highly efficient and accurate. However, casting the inverse problem into the CST framework is highly non-trivial. Although CST has been used to uncover the nodal interaction patterns for coupled oscillator networks or evolutionary games from time series [41] , [42] , [43] , the dynamics of epidemic propagation is typically highly stochastic with, for example, binary time series, rendering inapplicable the existing CST-based formulation. Further, despite the alternative sparsity enforcing regularizers and convex optimization used in ref. 44 to infer networks, CST has not been applied to reconstructing propagation networks, especially when the available time series are binary. The main accomplishment of this work is then the development of a scheme to implement the highly non-trivial transformation associated with the spreading dynamics in the paradigm of CST. Without loss of generality, we employ two prototypical models of epidemic spreading: classic susceptible-infected-susceptible (SIS) dynamics [13] and contact processes (CPs) [45] , [46] , on both model and real-world (empirical) networks. Inhomogeneous infection and recovery rates as representative characteristics of the natural diversity are incorporated into the diffusion dynamics to better mimic the real-world situation. We assume that only binary time series can be measured, which characterize the status of any node, infected or susceptible, at any time after the outbreak of the epidemic. The source that triggers the spreading process is assumed to be externally inaccessible (hidden). In fact, one may not even realize its existence from available time series. Our method enables, based on relatively small amounts of data, a full reconstruction of the epidemic spreading network with nodal diversity and successful identification of the immediate neighbouring nodes of the hidden source (thereby ascertaining its existence and uniquely specifying its connections to nodes in the network). The framework is validated with respect to different amounts of data generated from various combinations of the network structures and dynamical processes. High accuracy, high efficiency and applicability in a strongly stochastic environment with measurement noise and missing information are the most striking characteristics of our framework. Thus, broad applications can be expected in addressing significant problems such as targeted control of disease and rumour spreading. Compressed sensing The general problem that CST addresses is to reconstruct a vector X ε R N from linear measurements Y about X in the form where Y ε R M and Φ is an M × N matrix. The striking feature of CS is that the number of measurements can be much less than the number of components of the unknown vector, that is, M << N , insofar as X is sparse and the number of non-zero components in it is less than M . Accurate reconstruction can be achieved by solving the following convex-optimization problem [35] : where is the L 1 norm of X and the matrix Φ satisfies the restricted isometry property. Solutions to the convex optimization are now standard [35] , [36] , [37] , [38] , [39] , [40] . (More details of the CST can be found in Supplementary Note 1 .) Our goal is to develop a framework to cast the problem of reconstructing propagation networks into form (1). Reconstruction framework To present our framework in a transparent manner, we first consider the relatively simple case where there is no hidden source. Further, we assume that the disease starts to propagate from a fraction of the infected nodes. As we will see, based on this framework, it is feasible to locate any hidden source based solely on time series after outbreak of infection. The state of an arbitrary node i is denoted as S i , where Owing to the characteristic difference between the SIS dynamics and CP, we treat them separately (see Methods). For the SIS dynamics, the probability of an arbitrary node i being infected by its neighbors at time t is where λ i is the infection rate of i , a ij stands for the elements of the adjacency matrix ( a ij =1 if i connects to j and a ij =0 otherwise), S j ( t ) is the state of node j at t , and the superscript 01 denotes the change from susceptible state (0) to infected state (1). At the same time, the recovery probability of i is , where δ i is the recovery rate of node i and the superscript 10 denotes the transition from infected state to susceptible state. Equation (4) can be rewritten as If measurements at different times t = t 1 , t 2 , ···, t m are available, equation (5) can be written in the matrix form Y m × 1 = Φ m × ( N −1) · X ( N −1) × 1 , where Y contains at different t , Φ is determined by the state S j ( t ) of nodes except i , and X comprising the links and infection rates of i is sparse for a general network (see Methods). The main challenge here is that the infection probabilities at different times are not given directly from the time series of the nodal state. To develop a method to estimate the probability from the nodal states, we set a threshold Δ pertaining to the normalized Hamming distance between strings composed of S j ( t ) ( j≠i ) at different t to identify a base string at and a set of strings subject to the base. According to the law of large numbers, the probability can be estimated by the average over the state S i ( t +1) at all proper time. By setting another threshold Θ associated with the normalized Hamming distance, we can identify a set of base strings. This process finally gives rise to a set of reconstruction equations in the matrix form: where correspond to the time associated with m base strings and ‹·› denote the average over all satisfied t (see Methods). The vector Y m × 1 and the matrix Φ m × ( N −1) can then be obtained based solely on time series of nodal states and the vector X ( N −1) × 1 to be reconstructed is sparse, rendering applicable the CS framework. As a result, we can achieve exact reconstruction of all neighbours of node i from relatively small amounts of observation. In a similar manner the neighbouring vectors of all other nodes can be uncovered from time series, enabling a full reconstruction of the whole network by matching the neighboring sets of all nodes. For the CP dynamics, the infection probability of an arbitrary node i is given by where k i is the degree of the node i , and the recovery probability is (see Methods). In close analogy to the SIS dynamics, we have We then choose a series of base strings using a proper threshold Θ to establish a set of equations, expressed in the matrix form Y m × 1 = Φ m × ( N −1) · X ( N −1) × 1 (see Supplementary Note 2 ), where Φ has the same form as in equation (6), but Y and X are given by Our reconstruction framework based on establishing the vector Y and the matrix Φ is schematically illustrated in Fig. 1 . It is noteworthy that our framework can be extended to directed networks in a straightforward manner due to the feature that the neighbouring set of each node can be independently reconstructed. For instance, the neighbouring vector X can be defined to represent a unique link direction, for example, incoming links. Inference of the directed links of all nodes yields the full topology of the entire directed network. 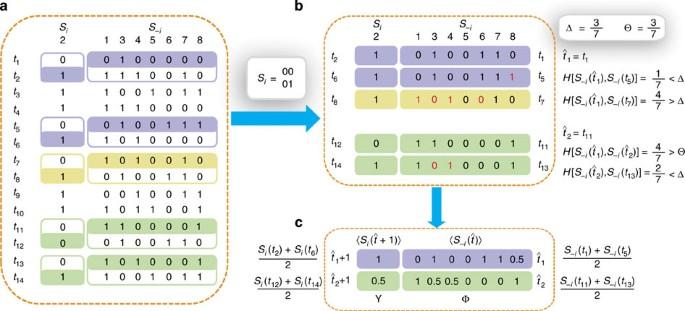Figure 1: Schematic illustration of building up Y and Φ from binary time series. (a) Fourteen snapshots of data at time instantst1−t14of eight nodes in a sample network, whereSiis the time series of node 2 andS−idenotes the strings of other nodes at different times. The neighbourhood of node 2 is to be reconstructed. Only the pairs 00 and 01 in the time series ofSi(i=2) and the correspondingS−icontain useful information about the network, as marked by different colours. (b) AsSi(t+1) is determined by the neighbours ofiandS−i(t), we sort outSi(t+1) andS−i(t) in the coloured sections of the time series ina. According to the threshold parametersΔ=3/7 and Θ=3/7, we calculate the normalized Hamming distance between each pair of stringsS−i(t), finding two base strings atandwith. We separate the coloured strings into two groups that are led by the two base strings, respectively. In each group, the normalized Hamming distancebetween the base string and other strings is calculated and the difference fromin each string is marked by red. Using parameterΔ, in the group led by,S−i(t5) andSi(t6) are preserved, because of. In contrast,S−i(t7) andSi(t8) are disregarded because. In the group led by, due to, the string is preserved. The two sets of remaining strings marked by purple and green can be used to yield the quantities required by the reconstruction formula. (Note that different base strings are allowed to share some strings, but for simplicity, this situation is not illustrated here. SeeSupplementary Note 3for a detailed discussion.) (c) The average valuesandused to extract the vectorYand the matrixΦin the reconstruction formula, where,,andbased on the remaining strings marked in different colours (see Methods for more details). CST can be used to reconstruct the neighbouring vectorXof node 2 fromYandΦfromY=Φ·X. Figure 1: Schematic illustration of building up Y and Φ from binary time series. ( a ) Fourteen snapshots of data at time instants t 1 − t 14 of eight nodes in a sample network, where S i is the time series of node 2 and S − i denotes the strings of other nodes at different times. The neighbourhood of node 2 is to be reconstructed. Only the pairs 00 and 01 in the time series of S i ( i =2) and the corresponding S − i contain useful information about the network, as marked by different colours. ( b ) As S i ( t +1) is determined by the neighbours of i and S − i ( t ), we sort out S i ( t +1) and S − i ( t ) in the coloured sections of the time series in a . According to the threshold parameters Δ =3/7 and Θ=3/7, we calculate the normalized Hamming distance between each pair of strings S − i ( t ), finding two base strings at and with . We separate the coloured strings into two groups that are led by the two base strings, respectively. In each group, the normalized Hamming distance between the base string and other strings is calculated and the difference from in each string is marked by red. Using parameter Δ , in the group led by , S − i ( t 5 ) and S i ( t 6 ) are preserved, because of . In contrast, S − i ( t 7 ) and S i ( t 8 ) are disregarded because . In the group led by , due to , the string is preserved. The two sets of remaining strings marked by purple and green can be used to yield the quantities required by the reconstruction formula. (Note that different base strings are allowed to share some strings, but for simplicity, this situation is not illustrated here. See Supplementary Note 3 for a detailed discussion.) ( c ) The average values and used to extract the vector Y and the matrix Φ in the reconstruction formula, where , , and based on the remaining strings marked in different colours (see Methods for more details). CST can be used to reconstruct the neighbouring vector X of node 2 from Y and Φ from Y = Φ·X . Full size image Reconstructing networks and infection and recovery rates To quantify the performance of our method in terms of the number of base strings (equations) for a variety of diffusion dynamics and network structures, we study the success rates for existent links (SRELs) and null connections (SRNCs), corresponding to non-zero and zero element values in the adjacency matrix, respectively. We impose the strict criterion that the network is regarded to have been fully reconstructed if and only if both success rates reach 100%. The sparsity of links makes it necessary to define SREL and SRNC separately. As the reconstruction method is implemented for each node in the network, we define SREL and SRNC on the basis of each individual node and the two success rates for the entire network are the respective averaged values over all nodes. We also consider the issue of trade-off in terms of the true positive rate (for correctly inferred links) and the false positive rate (for incorrectly inferred links). Here we assume that there is no hidden source and the spreading process starts from a fraction of infected nodes, and record the binary time series. 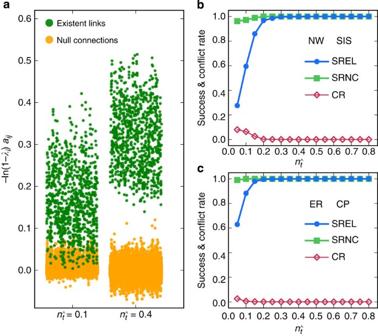Figure 2: Network reconstruction performance. (a) Element values ln(1−λi)aijof vectorXtimes −1 for different fractionof base strings for SIS dynamics. (b,c) Success rate (SREL and SRNC) and conflict rate (CR) of reconstruction as a function offor SIS dynamics on Newman–Watts (NW) small-world networks (b) and CP dynamics on Erdös–Rényi (ER) random networks (c). For the SIS dynamics, the parameters are Θ=0.25,Δ=0.45 and the infection and recovery ratesλiandδiare randomly distributed in the ranges (0.2, 0.4) and (0.4, 0.6), respectively. For the CP dynamics, the parameters are Θ=0.35,Δ=0.45 andλiandδiare randomly distributed in the ranges (0.7, 0.9) and (0.2, 0.4), respectively. The network sizeNis 200 with average node degree ‹k›=4. The results are obtained by ensemble averaging over ten independent realizations. The success rate is determined by setting a cut-off according toSupplementary Fig. 1aand the method described inSupplementary Note 4. Figure 2a shows the reconstructed values of the components of the neighbouring vector X of all nodes. Let be the number of base strings normalized by the network size N . For small values of , for example, , the values of elements associated with links and that associated with null connections (actual zeros in the adjacency matrix) overlap, leading to ambiguities in the identification of links. In contrast, for larger values of , for example, , an apparent gap emerges between the two groups of element values, enabling us to correctly identify all links by simply setting a cut-off within the gap (see Supplementary Fig. 1a and Supplementary Note 4 for a method to set the cut-off). The success rates (SREL and SRNC) as a function of for SIS and CP on both homogeneous and heterogeneous networks are shown in Fig. 2b,c , where we observe nearly perfect reconstruction of links insofar as exceeds a relatively small value—an advantage of compressed sensing. The exact reconstruction is robust in the sense that a wide range of values can yield nearly 100% success rates. Our reconstruction method is then effective for tackling real networks in the absence of any a priori knowledge about its topology. In particular, the existence of a clear gap in the reconstructed vector X represents a successful reconstruction for a real network. Figure 2: Network reconstruction performance. ( a ) Element values ln(1−λ i ) a ij of vector X times −1 for different fraction of base strings for SIS dynamics. ( b , c ) Success rate (SREL and SRNC) and conflict rate (CR) of reconstruction as a function of for SIS dynamics on Newman–Watts (NW) small-world networks ( b ) and CP dynamics on Erdös–Rényi (ER) random networks ( c ). For the SIS dynamics, the parameters are Θ=0.25, Δ =0.45 and the infection and recovery rates λ i and δ i are randomly distributed in the ranges (0.2, 0.4) and (0.4, 0.6), respectively. For the CP dynamics, the parameters are Θ=0.35, Δ =0.45 and λ i and δ i are randomly distributed in the ranges (0.7, 0.9) and (0.2, 0.4), respectively. The network size N is 200 with average node degree ‹ k ›=4. The results are obtained by ensemble averaging over ten independent realizations. The success rate is determined by setting a cut-off according to Supplementary Fig. 1a and the method described in Supplementary Note 4 . Full size image Note that a network is reconstructed through the union of all neighbourhoods, which may encounter ‘conflicts’ with respect to the presence/absence of a link between two nodes as generated by reconstruction centred at the two nodes. The conflicts would reduce the accuracy in the reconstruction of the entire network. To characterize the effects of edge conflicts, we study the consistency of mutual assessment of the presence or absence of link between each pair of nodes, as shown in Fig. 2b,c . We see that inconsistency arises for small values of but vanishes completely when the success rates reach 100%, indicating complete consistency among the mutual inferences of nodes and consequently guaranteeing accurate reconstruction of the entire network. Detailed results of success rates and trade-off measures with respect to a variety of model and real networks are displayed in Table 1 , Supplementary Figs 2 and 3 . and Supplementary Note 5 . Table 1 Performances of reconstruction and locating hidden source. Full size table Although the number of base strings is relatively small compared with the network size, we need a set of strings at different time with respect to a base string to formulate the mathematical framework for reconstruction. We study how the length of time series affects the accuracy of reconstruction. 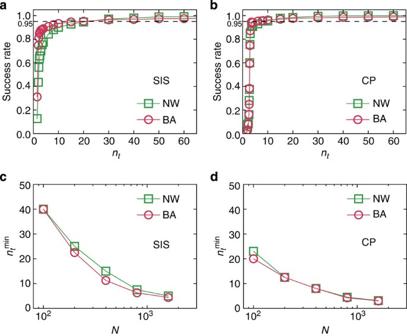Figure 3: Effect of the length of time series and network size. (a,b) Success rate as a function of the relative lengthntof time series for SIS (a) and CP (b) in combination with Newman–Watts (NW) and Barabási–Albert (BA) networks. The dashed lines represent 95% success rate. (c,d) the minimum relative lengththat assures at least 95% success rate as a function of the network sizeNfor SIS (c) and CP (d) dynamics on NW and BA networks. Here the success rate is the geometric average over SREL and SRNC. For SIS dynamics,λε(0.1, 0.3) andδε(0.2, 0.4). For CP dynamics,λε(0.7, 0.9) andδε(0.3, 0.5). Inaandb, the network sizeNis 500. The other parameters are the same as inFig. 2. Note thatnt≡t/N, wheretis the absolute length of time series, and, wheretminis the minimum absolute length of time series required for at least 95% success rate. Figure 3a,b show the success rate as a function of the relative length n t of time series for SIS and CP dynamics on both homogeneous and heterogeneous networks, where n t is the total length of time series from the beginning of the spreading process divided by the network size N . The results demonstrate that even for very small values of n t , most links can already be identified, as reflected by the high values of the success rate shown. Figure 3c,d show the minimum length required to achieve at least 95% success rate for different network sizes. For both SIS and CP dynamics on different networks, decreases considerably as N is increased. This seemingly counterintuitive result is due to the fact that different base strings can share strings at different times to enable reconstruction. In general, as N is increased, will increase accordingly. However, a particular string can belong to different base strings with respect to the threshold Δ, accounting for the slight increase in the absolute length of the time series (see Supplementary Fig. 4 and Supplementary Note 5 ) and the reduction in (see Supplementary Note 3 on the method to choose base and subordinate strings). The dependence of the success rate on the average node degree ‹ k › for SIS and CP on different networks has been investigated as well (see Supplementary Fig. 5 and Supplementary Note 5 ). The results in Figs 2 and 3 , Supplementary Figs 2–5 and Table 1 demonstrate the high accuracy and efficiency of our reconstruction method based on small amounts of data. Figure 3: Effect of the length of time series and network size. ( a , b ) Success rate as a function of the relative length n t of time series for SIS ( a ) and CP ( b ) in combination with Newman–Watts (NW) and Barabási–Albert (BA) networks. The dashed lines represent 95% success rate. ( c , d ) the minimum relative length that assures at least 95% success rate as a function of the network size N for SIS ( c ) and CP ( d ) dynamics on NW and BA networks. Here the success rate is the geometric average over SREL and SRNC. For SIS dynamics, λ ε(0.1, 0.3) and δ ε(0.2, 0.4). For CP dynamics, λ ε(0.7, 0.9) and δ ε(0.3, 0.5). In a and b , the network size N is 500. The other parameters are the same as in Fig. 2 . Note that n t ≡ t/N , where t is the absolute length of time series, and , where t min is the minimum absolute length of time series required for at least 95% success rate. Full size image In practice, noise is present and it is also common for time series from certain nodes to be missing, and it is necessary to test the applicability of our method in more realistic situations. 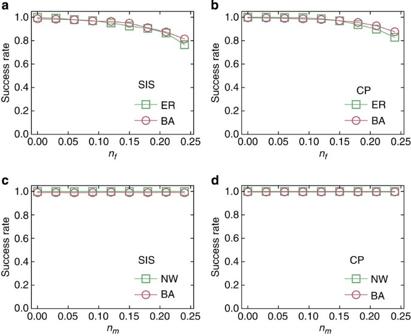Figure 4: Reconstruction against noise and inaccessible nodes. (a,b) Success rate as a function of the fractionnfof the flipped states induced by noise in time series for SIS (a) and CP (b) dynamics on Erdös–Rényi (ER) and Barabási–Albert (BA) networks. (c,d) Success rate as a function of the fractionnmof nodes that are externally inaccessible for SIS (c) and CP (d) dynamics on NW and BA networks. The network sizeNis 500 and ‹k›=4. The other parameters are the same as inFig. 2. Figure 4a,b show the dependence of the success rate on the fraction n f of states in the time series that flip due to noise for SIS and CP dynamics on two types of networks. We observe that the success rates are hardly affected, providing strong evidence for the applicability of our reconstruction method. For example, even when 25% of the nodal states flip, we can still achieve about 80% success rates for both dynamical processes and different network topologies. Figure 4c,d present the success rate versus the fraction n m of unobservable nodes, the states of which are externally inaccessible. We find that the high success rate remains mostly unchanged as n m is increased from 0 to 25%, a somewhat counterintuitive but striking result. The high degree of robustness against the limit to accessing nodal states is elaborated further in Supplementary Fig. 6 and Supplementary Note 5 . We find that, in general, missing information can affect the reconstruction of the neighbouring vector, as reflected by the reduction of the gap between the reconstructed values associated with actual links and null connections. However, even for high values of n m , for example, n m =0.3, there is still a clear gap, indicating that a full recovery of all links is achievable. We have also found that our method is robust against inaccurately specified diffusion processes with fluctuation in infection rates (see Supplementary Fig. 7 and Supplementary Note 5 ). Taken together, the high accuracy, efficiency and robustness against noise, missing information and inaccurately modelling of real dynamical processes provide strong credence for the validity and power of our framework for binary time-series-based network reconstruction. Figure 4: Reconstruction against noise and inaccessible nodes. ( a , b ) Success rate as a function of the fraction n f of the flipped states induced by noise in time series for SIS ( a ) and CP ( b ) dynamics on Erdös–Rényi (ER) and Barabási–Albert (BA) networks. ( c , d ) Success rate as a function of the fraction n m of nodes that are externally inaccessible for SIS ( c ) and CP ( d ) dynamics on NW and BA networks. The network size N is 500 and ‹ k ›=4. The other parameters are the same as in Fig. 2 . Full size image Having reconstructed the network structure, we can estimate the infection and recovery rates of individuals to uncover their diversity in immunity. This is an essential step to implement target vaccination strategy in a population or on a computer network to effectively suppress/prevent the spreading of virus at low cost, as a large body of literature indicates that knowledge about the network structure and individual characteristics is sufficient for controlling the spreading dynamics [47] , [48] , [49] , [50] . Here we offer an effective method to infer the individuals’ infection rates λ i based solely on the binary time series of the nodal states after an outbreak of contamination. (To our knowledge, there was no prior work addressing this critical issue.) In particular, after all links have been successfully predicted, λ i can be deduced from the infection probabilities that can be approximated by the corresponding infection frequencies (see Methods). These probabilities depend on both λ i and the number of infected neighbours. The reproduced infection rates λ i of individuals for both SIS and CP dynamics on different networks are in quite good agreement with the true values with small prediction errors (see Supplementary Fig. 8 and Supplementary Note 6 ). Results from a comprehensive error analysis are listed in Table 1 , where the uniformly high accuracy validates our method. The inhomogeneous recovery rates δ i of nodes can be predicted from the binary time series in a more straightforward way, because δ i do not depend on the nodal connections (see Supplementary Fig. 9 and Supplementary Note 6 ). Thus, our framework is capable of predicting characteristics of nodal diversity in terms of degrees, and infection and recovery rates based solely on binary time series of nodal states. Locating the hidden source of propagation We assume that a hidden source exists outside the network but there are connections between it and some nodes in the network. In practice, the source can be modelled as a special node that is always infected. Starting from the neighbourhood of the source, the infection originates from the source and spreads all over the network. We collect a set of time series of the nodal states, except the hidden source (see Methods). The basic idea of ascertaining and locating the hidden source is based on missing information from the hidden source when attempting to reconstruct the network. In particular, to reconstruct the connections belonging to the immediate neighbourhood of the source accurately, time series from the source are needed to generate the matrix Φ and the vector Y . However, as the source is hidden, no time series from it are available, leading to reconstruction inaccuracy and, consequently, anomalies in the predicted link patterns of the neighbouring nodes. It is then possible to detect the neighbourhood of the hidden source by identifying any abnormal connection patterns [51] , which can be accomplished by using different data segments. If the inferred links of a node are stable with respect to different data segments, the node can be deemed to have no connection with the hidden source; otherwise, if the result of inferring a node’s links varies significantly with respect to different data segments, the node is likely to be connected to the hidden source. The s.d. of the predicted results with respect to different data segments can be used as a quantitative criterion for the anomaly. Once the neighbouring set of the source is determined, the source is then precisely located topologically. 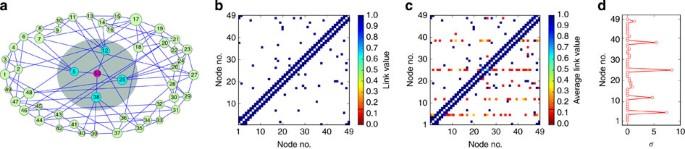Figure 5: Locating an external hidden source from time series. (a) Hidden source treated as a special node (in red) is connected to four nodes in the network (blue). The time series of other nodes except the source (number 50) after the outbreak of an epidemic are assumed to be available. (b) True adjacency matrix of the NW network with identical link weights to facilitate a comparison with the reconstructed adjacency matrix. (c) Reconstructed adjacency matrix from a number of segments in time series. The four neighbouring nodes of the source are predicted to be densely linked to other nodes, as indicated by the average value of the elements in the four rows corresponding to these nodes. (d) Structural varianceσof each node. The four neighbouring nodes of the source exhibit much larger values ofσthan those from the other nodes, providing unequivocal evidence that they belong to the immediate neighbourhood of the hidden source. Figure 5 presents an example, where a hidden source is connected with four nodes in the network ( Fig. 5a ), as reflected in the network adjacency matrix ( Fig. 5b ). We implement our reconstruction framework on each accessible node by using different sets of data in the time series. For each data set, we predict the neighbours of all nodes and generate an adjacency matrix. Averaging over the elements corresponding to each location in all the reconstructed adjacency matrices, we obtain Fig. 5c , in which each row corresponds to the mean number of links in a node’s neighbourhood. The inferred links of the immediate neighbours of the hidden source exhibit anomalies. To quantify the anomalies, we calculate the structural s.d. σ from different data segments, where σ associated with node i is defined through the i th row in the adjacency matrix as Figure 5: Locating an external hidden source from time series. ( a ) Hidden source treated as a special node (in red) is connected to four nodes in the network (blue). The time series of other nodes except the source (number 50) after the outbreak of an epidemic are assumed to be available. ( b ) True adjacency matrix of the NW network with identical link weights to facilitate a comparison with the reconstructed adjacency matrix. ( c ) Reconstructed adjacency matrix from a number of segments in time series. The four neighbouring nodes of the source are predicted to be densely linked to other nodes, as indicated by the average value of the elements in the four rows corresponding to these nodes. ( d ) Structural variance σ of each node. The four neighbouring nodes of the source exhibit much larger values of σ than those from the other nodes, providing unequivocal evidence that they belong to the immediate neighbourhood of the hidden source. Full size image where j denotes the column, represents the element value in the adjacency matrix inferred from the k th group of the data, is the mean value of a ij and g is the number of data segments. Applying equation (10) to the reconstructed adjacency matrices gives the results in Fig. 5d , where the values of σ associated with the immediate neighbouring nodes of the hidden source are much larger than those from others (which are essentially zero). A cut-off value can be set in the distribution of σ i to identify the immediate neighbours of the hidden source (see Supplementary Fig. 1b and Supplementary Note 4 ). The performance of locating hidden source by means of the trade-off measures (true positive rate versus false positive rate) are displayed in Table 1 . We have developed a general framework to reconstruct complex propagation networks on which epidemic spreading takes place from binary time series. Our paradigm is based on compressed sensing, is completely data-driven and practically significant for controlling epidemic spreading through targeted vaccination. Both theoretically and practically, our framework can be used to address the extremely challenging problem of reconstructing the intrinsic interacting patterns of complex stochastic systems based on small amounts of polarized time series. The key to success of our method lies in our development of a novel class of transformation, allowing the network inference problem to be converted to the problem of sparse signal reconstruction, which can then be solved by the standard compressed-sensing algorithm. The accuracy and efficiency of our framework in uncovering the network structure, the natural diversity in the nodal characteristics, and any hidden source are guaranteed by the CST with rigorous proof for low-data requirement and convergence to optimal solution. The feasibility of our framework has been demonstrated using a large number of combinations of epidemic processes and network structures, where in all cases highly accurate reconstruction is achieved. Our approach opens up a new avenue towards fully addressing the inverse problem in complex stochastic systems in a highly efficient manner, a fundamental stepping stone towards understanding and controlling complex dynamical systems in general. We have focused on two types of spreading dynamics, SIS and CP, where an infected individual can recover and becomes susceptible again. In this regard, even if an outbreak occurs, control strategy such as targeted vaccination or quarantine can be helpful to eliminate the virus eventually. A main purpose of our work is to identify the key individuals in the network to implement target control and to locate the source of infection to isolate it so as to prevent recurrent infection in the future. Although for any spreading dynamics, the most effective way to prevent a large-scale outbreak is to implement control during the early stage, this may be impractical in many situations. If we miss the early stage, which is possible especially in complex networks where the epidemic threshold can be near zero, to be able to reconstruct the spreading network is of tremendous value. Besides disease spreading, our framework is applicable to rumour or information spreading. In this case, identifying the source of rumour is important, a problem that our framework is capable of solving. Our work raises a number of questions to further and perfect the theoretical and algorithmic development of reconstructing complex dynamical systems. For example, if partial knowledge about the network structure is available, the information can be incorporated into our framework to further reduce the required data amount. Moreover, for non-Markovian spreading processes, our current reconstruction framework may fail. This raises the need to develop new and more general approaches. Nevertheless, our theory, due to its generality and applicability to various types of inhomogeneous interactions, can be applied to networks of networks or interdependent networks, in which there may be different spreading patterns associated with distinct layers or components. Taken together, our results provide strong credence to the proposition that complex networks can be fully decrypted from measurements, even when stochastic disturbance and hidden sources are present. This can offer a deeper understanding of complex systems in general and significantly enhance our ability to control them based on, for example, the recently developed controllability theory of complex networks [52] , [53] , [54] , [55] , [56] , [57] , [58] . Spreading processes The SIS model is a classic epidemic model that has been used frequently to study a variety of spreading behaviours in social and computer networks. Each node of the network represents an individual and links are connections along which infection can propagate to others with certain probability. At each time step, a susceptible node i in state 0 is infected with rate λ i if it is connected to an infected node in state 1. If i connects to more than one infected neighbour, the infection probability P 01 is given by equation (4). At the same time, infected nodes are continuously recovered to be susceptible at the rates δ i . The CP model has been used extensively to describe, for example, the spreading of infection and competition of animals over a territory, where λ i is determined by equation (7). The main difference between SIS and CP dynamics lies in the influence on a node’s state from its vicinity. In both SIS and CP dynamics, λ i and δ i depend on the individuals’ immune systems and are selected from a uniform distribution characterizing the natural diversity (see Supplementary Note 7 for details of numerical simulations). Moreover, a hidden source is regarded as infected for all time. Mathematical formulation of reconstruction based on CST For SIS dynamics, suppose measurements at a sequence of times t = t 1 , t 2 , ···, t m are available. equation (5) leads to the following matrix form Y m × 1 = Φ m × ( N −1) · X ( N −1) × 1 : where the vector X ( N −1) × 1 contains all possible connections between node i and all other nodes, and it is sparse for a general complex network. We see that if the vector Y m × 1 and the matrix Φ m × ( N −1) can be constructed from time series, X ( N −1) × 1 can then be solved by using CST. The main challenge here is that the infection probabilities at different times are not given directly by the time series of the nodal states. To devise a heuristic method to estimate the probabilities, we assume that the neighbouring set Γ i of the node i is known. The number of such neighbouring nodes is given by k i , the degree of node i and their states at time t can be denoted as To approximate the infection probability, we use S i ( t )=0 so that at t +1, the node i can be infected with certain probability. In contrast, if S i ( t )=1, S i ( t +1) is only related with the recovery probability δ i . Hence, we focus on the S i ( t )=0 case to derive . If we can find two time instants: t 1 , t 2 ε T ( T is the length of time series), such that S i ( t 1 )=0 and S i ( t 2 )=0, we can then calculate the normalized Hamming distance between and , where the normalized Hamming distance between two strings of equal length is defined as ratio of the number of positions with different symbols between them and the length of string. If , we can regard the states at the next time step, S i ( t 1 +1) and S i ( t 2 +1), as i.i.d Bernoulli trials. In this case, using the law of large numbers, we have A more intuitive understanding of (equation (12)) is that if the states of i ’s neighbours are unchanged, the fraction of times of i being infected by its neighbours over the entire time period will approach the actual infection probability . Note, however, that the neighbouring set of i is unknown and to be inferred. A strategy is then to artificially enlarge the neighbouring set to include all nodes in the network, except i . In particular, we denote If H [ S − i ( t 1 ), S − i ( t 2 )]=0, the condition will be ensured. Consequently, due to the nature of i.i.d Bernoulli trials, from the law of large numbers, we have Hence, the infection probability of a node at can be evaluated by averaging over its states associated with zero-normalized Hamming distance between the strings of other nodes at some time associated with . In practice, to find two strings with absolute zero-normalized Hamming distance is unlikely. We thus set a threshold Δ so as to pick the suitable strings to approximate the law of large numbers, that is where serves as a base for comparison with S − i ( t ) at all other times and . As is not exactly zero, there is a small difference between and . We thus consider the average of for all t ν to obtain , leading to the right-hand side of equation (14). We denote and . To reduce the error in the estimation, we implement the average on S − i ( t ) over all selected strings through equation (14). The averaging process is with respect to the nodal states S j , j ,≠ i ( t ) on the right-hand side of the modified dynamical equation (5). Specifically, averaging over time t restricted by equation (14) on both sides of equation (5), we obtain . If λ i is small with insignificant fluctuations, we can approximately have (see Supplementary Fig. 10 and Supplementary Note 8 ), which leads to . Substituting by , we finally get Although the above procedure yields an equation that bridges the links of an arbitrary node i with the observable states of the nodes, a single equation does not contain sufficient structural information about the network. Our second step is then to derive a sufficient number of linearly independent equations required by CST to reconstruct the local connection structure. To achieve this, we choose a series of base strings at a number of time instants from a set denoted by T base , in which each pair of strings satisfy where and correspond to the time instants of two base strings in the time series and Θ is a threshold. For each string, we repeat the process of establishing the relationship between the nodal states and connections, leading to a set of equations at different values of in equation (15), as described in the matrix form (equation (6)). See Supplementary Fig. 11, 12 and Supplementary Note 8 for the dependence of success rate on threshold Δ and Θ for SIS and CP dynamics in combination with four types of networks. Inferring inhomogeneous infection rates The values of the infection rate λ i of nodes can be inferred after the neighbourhood of each node has been successfully reconstructed. The idea roots in the fact that the infection probability of a node approximated by the frequency of being infected calculated from time series is determined both by its infection rate and by the number of infected nodes in its neighbourhood. To provide an intuitive picture, we consider the following simple scenario in which the number of infected neighbours of node i does not change with time. In this case, the probability of i being infected at each time step is fixed. We can thus count the frequency of the 01 and 00 pairs embedded in the time series of i . The ratio of the number of 01 pairs over the total number of 01 and 00 pairs gives approximately the infection probability. The infection rate can then be calculated by using equations (4) and (7) for the SIS and CP dynamics, respectively. In a real-world situation, however, the number of infected neighbours varies with time. The time-varying factor can be taken into account by sorting out the time instants corresponding to different numbers of the infected neighbours, and the infection probability can be obtained at the corresponding time instants, leading to a set of values for the infection rate whose average represents an accurate estimate of the true infection rate for each node. To be concrete, considering all the time instants t ν associated with k I infected neighbors, we denote , ∀ t ν , and S i ( t ν )=0, where Γ i is the neighbouring set of node i , k I is the number of infected neighbours and represents the average infected fraction of node i with k I infected neighbours. Given , we can rewrite equation (4) by substituting for and for λ i , which yields . To reduce the estimation error, we average with respect to different values of k I , as follows: where Λ i denotes the set of all possible infected neighbours during the epidemic process and denotes the number of different values of k I in the set. Analogously, for CP, we can evaluate from equation (7) by where is the node degree of i . Insofar as all the links of i have been successfully reconstructed, can be obtained from the time series in terms of the satisfied S i ( t ν +1), allowing us to infer via equations (17) and (18). Note that the method is applicable to any type of networks insofar as the network structure has been successfully reconstructed. Networks analysed Model networks and real networks we used are described in Supplementary Note 10 and Table 1 . How to cite this article: Shen, Z. et al . Reconstructing propagation networks with natural diversity and identifying hidden sources. Nat. Commun. 5:4323 doi: 10.1038/ncomms5323 (2014).